Molecular mechanism of Mg2+-dependent gating in CorA CorA is the major transport system responsible for Mg 2+ uptake in bacteria and can functionally substitute for its homologue Mrs2p in the yeast inner mitochondrial membrane. Although several CorA crystal structures are available, the molecular mechanism of Mg 2+ uptake remains to be established. Here we use electron paramagnetic resonance spectroscopy, electrophysiology and molecular dynamic simulations to show that CorA is regulated by cytoplasmic Mg 2+ acting as a ligand and elucidate the basic conformational rearrangements responsible for Mg 2+ -dependent gating. Mg 2+ unbinding at the divalent cation sensor triggers a conformational change that leads to the inward motion of the stalk helix, which propagates to the pore-forming transmembrane helix TM1. Helical tilting and rotation in TM1 generates an iris-like motion that increases the diameter of the permeation pathway, triggering ion conduction. This work establishes the molecular basis of a Mg 2+ -driven negative feedback loop in CorA as the key physiological event controlling Mg 2+ uptake and homeostasis in prokaryotes. Magnesium (Mg 2+ ) is the most abundant divalent cation in biology [1] and is essential to all living cells as it participates in a myriad of key physiological and biochemical processes from enzymatic activity to genomic stability. In bacteria, Mg 2+ homeostasis is carried out by three molecularly distinct translocation systems, MgtA/B, MgtE and CorA [2] . CorA belongs to the GMN (Gly-Met-Asn) family and has been proposed to be one of the major Mg 2+ uptake pathway [3] . Since the discovery of the CorA gene [4] , the pioneering work of Maguire and colleagues [5] , [6] , [7] using in vivo radiotracer measurement have provided the functional and genetic basis for its role in bacteria. The structures of CorA from Thermotoga maritima offered the first structural template to understand Mg 2+ permeation and transport [8] , [9] , [10] . The GMN family is characterized by relatively low-sequence conservation and several reports have suggested conflicting transport mechanisms for Tm CorA [11] , [12] . However, electrophysiological data show that CorA-driven Mg 2+ translocation involves a channel-like mechanism where the inwardly biased electrochemical gradient serves as the main driving force for Mg 2+ permeation [13] . So far, the available Tm CorA structures have shown the presence of a density commensurate with a divalent cation at the GMN signature sequence and another ion density located in the cytoplasmic end of the pore [14] , [15] . This leaves a long (~30 Å) narrow pathway without apparent coordination sites for permeating ions, providing no obvious insights in regard to the molecular basis of Mg 2+ selectivity and permeation for Tm CorA and other members of the GMN family. Molecular dynamic (MD) simulations and electrostatic calculations have suggested that the present set of divalent-bound crystal structures represents a non-conductive state [16] , [17] . A recent structure of a distant Tm CorA homologue from Methanocaldococcus jannaschii has revealed the first structural glimpses into the determinants of Mg 2+ selectivity. An electron density asymmetrically positioned in the outer mouth of the pore has been interpreted as Mg 2+ with its first water shell [18] . Interestingly, this new structure points to a putative role for residue Asn314 at the GMN signature sequence in selectivity. A recent Tm CorA structure shows a similar density coordinated by the same residue triad, suggesting that Mg 2+ coordination by the GMN signature sequence is a common motif within the family [14] . Using a combination of electrophysiology and mutagenesis, we have shown that the GMN motif likely participates in the formation of a high-affinity Mg 2+ -binding site that defines CorA selectivity via a knock-in knockout repulsion mechanism [13] . Indeed, as derived from the present set of structures, such a long and seemingly inhospitable pore (devoid of ions) has been considered as one of the key arguments, suggesting that widespread conformational rearrangements must take place to allow Mg 2+ permeation [16] , [17] . However, attempts to stabilize the conductive conformation of CorA by eliminating divalent ions in the crystallization matrix have been unsuccessful, and the quest for a conductive conformation remains ongoing. Here we have used electrophysiological and spectroscopic approaches to address two fundamental questions regarding CorA-driven Mg 2+ translocation: (i) the nature and location of the gate that opens the permeation pathway, and (ii) the molecular movements that underlie Mg 2+ -driven gating. Using a large set of cysteine mutants targeted to the two transmembrane (TM) segments and the entire stalk helix, we show that binding of Mg 2+ to the intracellular divalent cation sensor triggers channel closing. Comparison of individual electron paramagnetic resonance (EPR) parameters from the complete set of spin-labelled (SL) mutants provided information on probe dynamics, solvent accessibility and intersubunit distances in the conformationally trapped states. These data, combined with existing crystal structures and computational approaches, were used to depict the structural rearrangements associated with Mg 2+ -dependent gating and to generate three-dimensional (3D) models of CorA in its putative conductive conformation. CorA is gated by intracellular Mg 2+ In vivo transport measurements of CorA show that shortly after a rapid Mg 2+ uptake, its intracellular concentration remains steady, suggesting that the activity of CorA might be self-regulated [19] . Further, i n vitro studies have revealed a Mg 2+ -dependent protease susceptibility, a clear indication that Mg 2+ translocation through CorA must involve substantial structural rearrangements [10] , [14] , [20] . We have generated overexpression constructs that produce large Tm CorA-catalysed ionic currents in Xenopus oocytes [13] . This Mg 2+ inward current peaks within a few seconds (a reflection of the speed of the solution exchange) and spontaneously decays over the course of 15–20 min to a small (<5% of peak) steady-state current ( Fig. 1a ). The decay time constants are correlated with the current intensity and the nature of the permeant ion, leading us to suggest that internal Mg 2+ likely serves a dual role as both permeant ion and gating ligand for CorA ( Fig. 2 ). At high intracellular Mg 2+ concentration (>5 mM), CorA-catalysed currents are small or non-existent but as the intracellular concentration drops below 1–2 mM channel opening is triggered, supporting robust Mg 2+ inward currents. This was directly confirmed by using a cut-open oocyte setup where the local Mg 2+ concentration is tightly buffered and constantly perfused through a cannula positioned close to the membrane ( Fig. 1b ). Under those conditions, the inward current is abolished as a consequence of increasing internal Mg 2+ concentration with an apparent Mg 2+ affinity of 2.4 mM, which also corresponds to the physiological concentration in bacteria (2–3 mM) [21] . These conformational transitions are best fitted with the Hill number of 2 ( n H =2) and suggest a positive cooperativity for the Mg 2+ -driven gating transition ( Fig. 1f ). 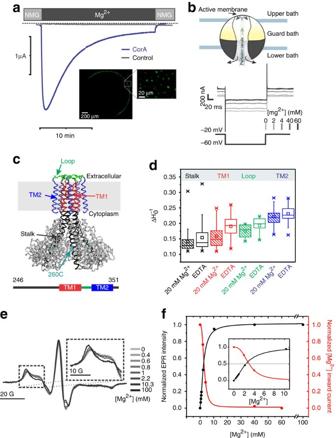Figure 1: CorA is gated by intracellular Mg2+. (a)TmCorA-specific Mg2+currents are recorded on a perfused two-electrode voltage clamp setup. The representative traces are recorded at a constant −60 mV for aXenopusoocyte injected with mRNA coding forTmCorA and an oocyte injected with water (control). The currents are recorded with constant external perfusion changing from a divalent-free solution (N-methyl glucamine) to a 20 mM Mg2+buffer. The inset represents a confocal microscopy image of an oocyte injected with the YFP-TmCorA fusion construct. (b) The internal perfusion cut-open oocyte voltage clamp setup used for this experiment is schematized in the upper panel. The representative trace is shown in the lower panel for each internal buffer tested. (c) Schematic representation of the cysteine scan used for this work. The covered sequence is shown in black red, green and blue. (d) Statistical representation of the probe mobility parameterfor the different secondary structure elements. Boxes are the 25–75% with the median as horizontal line, the little squares show the mean values, and the asterisks show the 1–99% using the same colour code as for panelc. (e) CW-EPR spectra recorded for the Q260C-SL mutant in presence of various Mg2+concentrations. (f) Titration plot of the normalized Mg2+-dependent currents superimposed with Mg2+conformational transition recorded by CW-EPR. Both plots were fitted by a Hill equation. The inset is a magnification of the low concentration range. Figure 1: CorA is gated by intracellular Mg 2+ . ( a ) Tm CorA-specific Mg 2+ currents are recorded on a perfused two-electrode voltage clamp setup. The representative traces are recorded at a constant −60 mV for a Xenopus oocyte injected with mRNA coding for Tm CorA and an oocyte injected with water (control). The currents are recorded with constant external perfusion changing from a divalent-free solution ( N -methyl glucamine) to a 20 mM Mg 2+ buffer. The inset represents a confocal microscopy image of an oocyte injected with the YFP- Tm CorA fusion construct. ( b ) The internal perfusion cut-open oocyte voltage clamp setup used for this experiment is schematized in the upper panel. The representative trace is shown in the lower panel for each internal buffer tested. ( c ) Schematic representation of the cysteine scan used for this work. The covered sequence is shown in black red, green and blue. ( d ) Statistical representation of the probe mobility parameter for the different secondary structure elements. Boxes are the 25–75% with the median as horizontal line, the little squares show the mean values, and the asterisks show the 1–99% using the same colour code as for panel c . ( e ) CW-EPR spectra recorded for the Q260C-SL mutant in presence of various Mg 2+ concentrations. ( f ) Titration plot of the normalized Mg 2+ -dependent currents superimposed with Mg 2+ conformational transition recorded by CW-EPR. Both plots were fitted by a Hill equation. The inset is a magnification of the low concentration range. 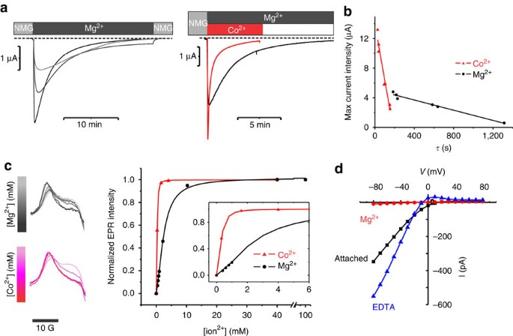Figure 2: Divalent cations are both charge carriers and gating factors. (a) Representative traces of Mg2+currents are recorded in CorA-expressingX. laevisoocytes clamped at −60 mV. Right trace; Mg2+(20 mM) current traces are in black and the Co2+(20 mM) current is in red. (b) Correlation between peak currents and inhibition time constant (single exponential decay fit). The results are plotted in black and red for Mg2+and Co2+as charge carriers, respectively. (c) Low-field region of X-band CW-EPR spectra of CorA SL at position 260C titrated by Co2+and Mg2+are shown. The resulting titration plots are displayed using the same colour code for the ions. A magnification of the lower concentration range is displayed in the inset. The plots were fitted with a Hill equation and the apparent affinity is 2.4 mM for Mg2+and 0.29 mM for Co2+. (d) I/V curve of excised patch inside in the inside out configuration when the cytoplasmic domain is bathed in presence of divalent chelating compound or a 10-mM concentration of Mg2+. Full size image Figure 2: Divalent cations are both charge carriers and gating factors. ( a ) Representative traces of Mg 2+ currents are recorded in CorA-expressing X. laevis oocytes clamped at −60 mV. Right trace; Mg 2+ (20 mM) current traces are in black and the Co 2+ (20 mM) current is in red. ( b ) Correlation between peak currents and inhibition time constant (single exponential decay fit). The results are plotted in black and red for Mg 2+ and Co 2+ as charge carriers, respectively. ( c ) Low-field region of X-band CW-EPR spectra of CorA SL at position 260C titrated by Co 2+ and Mg 2+ are shown. The resulting titration plots are displayed using the same colour code for the ions. A magnification of the lower concentration range is displayed in the inset. The plots were fitted with a Hill equation and the apparent affinity is 2.4 mM for Mg 2+ and 0.29 mM for Co 2+ . ( d ) I/V curve of excised patch inside in the inside out configuration when the cytoplasmic domain is bathed in presence of divalent chelating compound or a 10-mM concentration of Mg 2+ . Full size image We have investigated the conformation of liposome-reconstituted CorA in the following two different experimental conditions: without Mg 2+ (apo form) and at saturating Mg 2+ concentrations (20 mM). Continuous wave EPR spectroscopy (CW-EPR) was used to determine the spectral properties of for more than 100 SL cysteine mutants ( Fig. 1c ). Figure 1d reports the global change in probe mobility ( ) [22] in four different regions of CorA, clearly showing widespread structural rearrangement associated with the presence of Mg 2+ . From this large data set, position 260 displays one of the largest spectral changes between the apo and Mg 2+ -bound forms of CorA, making it an ideal reporter to establish the Mg 2+ dependence of the conformational changes in CorA ( Fig. 1d,e ). Assessed from the SL mobility, the overall Mg 2+ dependence of the structural changes is similar to that obtained for the inhibitory gating measured by perfused cut-open oocyte voltage clamp ( Fig. 1f ). Equivalent conformational transitions were observed in the absence of a lipid bilayer, implying that the Mg 2+ -dependent structural changes are self-contained, with no direct participation of the lipid bilayer ( Supplementary Fig. 1 ). We conclude that the Mg 2+ -driven deactivation of Mg 2+ currents ( Fig. 1a,b ) and the Mg 2+ -induced conformational transitions observed by EPR ( Fig. 1e ) are a reflection of the very same molecular events that underlie Mg 2+ -dependent gating in CorA. This conclusion is further supported by several pieces of information that relate these time-dependent current changes to a fundamental property of CorA gating. First, when Mg 2+ current are increased by variation of the CorA expression levels, a concomitant acceleration in Mg 2+ current decay is observed ( Fig. 2a,b ). Second, other divalent cations such as Co 2+ are not only able to permeate CorA but also induce current decay with much faster kinetics than those obtained with Mg 2+ as charge carrier ( Fig. 2a,b ). Structural rearrangements can be followed as a function of Mg 2+ or Co 2+ concentrations and are best fitted by a classical Hill-binding model with an apparent affinity for Mg 2+ of K 0.5 =2.4 mM and for Co 2+ of K 0.5 =0.2 mM, both showing positive cooperativity ( n H =2) ( Fig. 2c ). The higher Co 2+ affinity detected by spectroscopy is consistent with the faster rate of inward current decays ( Fig. 2a,b ) and with previous Co 2+ -binding experiments, but is in the toxicity range of this cation that seems incompatible with a role of CorA as a regulator of Co 2+ homeostasis as previously proposed [11] . Third, excised patch clamp experiments show that exposure of the intracellular domain of CorA to millimolar concentrations of Mg 2+ leads to a reduction and, eventually, to the complete inhibition of the CorA-driven Mg 2+ currents. However, pre-exposing the cytoplasmic side to EDTA under the same experimental conditions consistently enhances Mg 2+ current amplitudes ( Fig. 2d ). We interpreted these phenomena to be the result of a self-regulatory mechanism, where an increase in the local Mg 2+ concentration on the intracellular side of the membrane saturates a CorA Mg 2+ -binding site, ultimately triggering channel closure. Under this scheme, the apo form of CorA is conductive and Mg 2+ binding triggers channel deactivation and stabilizes the non-conductive (closed) state of the channel. This mechanism where the charge carrier being also the gating factor fully supports the suggestion that Mg 2+ homeostasis in bacteria takes place through a Mg 2+ negative feedback loop [2] , [10] , [20] . The divalent cation sensor The crystal structures of Tm CorA obtained in a high concentration of divalent ions (Mg 2+ , Co 2+ and Ca 2+ ) point to the likely location of the divalent cation sensor [8] , [9] , [10] . A clear electron density was unequivocally assigned to divalent ions coordinated between two aspartate residues, Asp253 from one subunit and Asp89 from its adjacent subunit [8] ( Fig. 3a ). Mutating these residues alters the Mg 2+ -dependent protease digestion susceptibility, implying that these residues might be involved in magnesium sensing [10] . Using both spectroscopic and electrophysiological approaches, we find that disrupting the contribution of individual components of this putative site markedly alters Mg 2+ binding. Replacing Asp253 or Asp89 by a lysine abolishes the Mg 2+ -dependent conformational transition observed at position Asn260 (near the divalent-binding site) by EPR spectroscopy ( Fig. 3b ). Also, given the similarities with the EPR spectra of D89K-D253, D89-D253K and Mg 2+ -bound wild-type (WT) CorA (again at position Asn260), the conformational equilibrium of the divalent-binding site mutant seems to be biased towards the closed state. This observation is supported by a moderate loss of function phenotype in a cell complementation assay [20] . Based on this observation, we argue that the conformational motions monitored at position 260 directly correlate with the presence of Mg 2+ at the divalent-binding site. Oocytes injected with the D253K construct can still generate a CorA-specific Mg 2+ inward current, but in contrast to the WT channel they do not exhibit a time-dependent decay ( Fig. 3c ), and thus facilitate permeation studies [13] . This result is the most direct demonstration that the interacting pair Asp253-Asp89 acts as an important component of the divalent cation sensor in CorA. This divalent sensor presumably probes the intracellular concentration of Mg 2+ and triggers an allosteric conformational wave that leads to channel closure as Mg 2+ reaches above its physiological level. Interestingly, MgtE also seems to operate with a self-regulated mechanism despite any structural nor sequence similarity to CorA [23] , [24] . 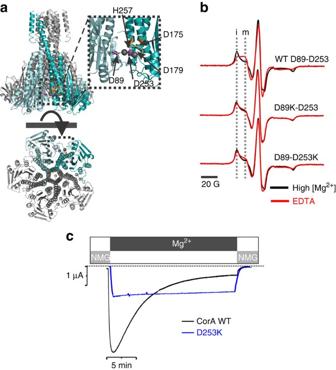Figure 3: The divalent cation sensor. (a) Close-up view of the putative regulatory Mg2+-binding domain revealed by the crystal structure. (b) EPR spectra of the Q260C-SL mutant recorded in presence of 20 mM Mg2+shown in black and in absence of divalent cation shown in red. The experiments were repeated in the background of the WT protein, D89K and D253K mutation. The immobile (i) and mobile (m) components of the low-field spectra are highlighted by two vertical dash lines. (c) Representative macroscopic current traces recorded for WT CorA and D253K are shown in black and blue, respectively. Figure 3: The divalent cation sensor. ( a ) Close-up view of the putative regulatory Mg 2+ -binding domain revealed by the crystal structure. ( b ) EPR spectra of the Q260C-SL mutant recorded in presence of 20 mM Mg 2+ shown in black and in absence of divalent cation shown in red. The experiments were repeated in the background of the WT protein, D89K and D253K mutation. The immobile (i) and mobile (m) components of the low-field spectra are highlighted by two vertical dash lines. ( c ) Representative macroscopic current traces recorded for WT CorA and D253K are shown in black and blue, respectively. Full size image Gating involves expansion of the intracellular cavity To gain further insight into the CorA-gating mechanism, we carried out a complete characterization of the environmental properties of SLs attached to cysteine residues located along the long stalk helix (residues 246–293), the pore-forming TM1 helix (residues 294–314), the extracellular loop (residues 315–325) and the lipid-facing TM2 helix (residues 326–348). We analysed three structural parameters from CW-EPR spectral properties such as probe mobility ( ) that reflects the conformational flexibility [22] (larger values imply higher motional freedom); collision with NiEDDA, an indicator of water exposure; and collision with O 2 that monitors lipid exposure [25] , [26] ( Fig. 4a ). Measurements were carried out in high Mg 2+ , which should favour the closed conformation, and in the nominal absence of Mg 2+ (or other divalent ions), which should populate the open state of CorA. 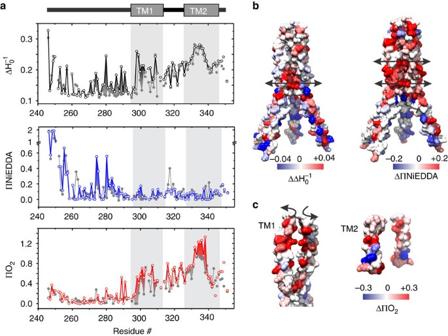Figure 4: Probe environmental parameters and structural rearrangement associated with gating. (a) Probe mobility, NiEDDA accessibility and O2accessibly values were plotted against the residue number for two experimental conditions: 20 mM Mg2+and no Mg2+. The values for sample recorded in presence of Mg2+(closed state) are shown in grey closed circle, whereas the values obtained for CorA in its open conformation are shown as coloured open circles. (b) The differential mobility values between the open and the closed conformation were colour coded from red to blue and mapped on the crystal structure of CorA. For clarity purposes, only the stalk helix and Tm1 are shown and one subunit has been removed. Similar representation is shown on the right side for the differential values in NiEDDA colliding agent. (c) Differential O2accessibility are colour scaled and mapped on TM1 (left panel) and TM2 (right panel). Only two subunits are shown for clarity purposes. Figure 4: Probe environmental parameters and structural rearrangement associated with gating. ( a ) Probe mobility, NiEDDA accessibility and O 2 accessibly values were plotted against the residue number for two experimental conditions: 20 mM Mg 2+ and no Mg 2+ . The values for sample recorded in presence of Mg 2+ (closed state) are shown in grey closed circle, whereas the values obtained for CorA in its open conformation are shown as coloured open circles. ( b ) The differential mobility values between the open and the closed conformation were colour coded from red to blue and mapped on the crystal structure of CorA. For clarity purposes, only the stalk helix and Tm1 are shown and one subunit has been removed. Similar representation is shown on the right side for the differential values in NiEDDA colliding agent. ( c ) Differential O 2 accessibility are colour scaled and mapped on TM1 (left panel) and TM2 (right panel). Only two subunits are shown for clarity purposes. Full size image Comparing solvent accessibility and probe mobility revealed a series of marked Mg 2+ -driven structural changes in CorA ( Fig. 4b ). In the Apo form, residues from the stalk helix forming the inner cavity of the intracellular funnel show increased mobility and NiEDDA accessibility (ПNiEDDA), particularly for residues Gly274, Leu280, Val283 and Thr287. Differences in ПNiEDDA between the apo- and Mg 2+ -bound states mapped onto the crystal structure of Tm CorA (closed state; Fig. 4b ) show that the major increases in ПNiEDDA and take place inside the funnel cavity (arrows). These results point to a widening of the inner funnel cavity as Mg 2+ is removed from its regulatory domain. Consistent with the fairly large cavity expansion, the sharp increase in probe mobility seems to occur in both faces of the helix as a result of reduced helical packing in the open (apo) conformation. Given the size of NiEDDA compared with a water molecule, we anticipate that the functionally relevant magnitudes of the conformational transitions extend further beyond the mapped increases and represent a widespread reorientation of the permeation pathway as a whole. This is supported by significant changes in the O 2 accessibility (ПO 2 ) along the TM helices ( Fig. 4d ). The relatively large increase in ПO 2 profile along pore-facing residue in TM1 indicates a relative reorientation of this helix ( Fig. 4c ). These changes are compatible with the unbending of helix TM1, ultimately leading to an increase in the diameter of the permeation pathway. The very high ПO 2 values reported for TM2 indicate that the intimate contact between TM1 and TM2 are disrupted in the open conformation. Conformational changes were also observed for TM1 as evaluated from the collision to the DOGS-NTA[Ni(II)] lipid, a collisional agent that reports on interfacial accessibility ( Supplementary Fig. 2 ). This strongly supports a sizable and widespread structural rearrangement upon Mg 2+ -driven gating that appears to be larger than the relatively modest radial and lateral tilts of the stalk helix α7 recently reported [14] . Inner motion of the stalk helix leads to pore opening As expected from a radially symmetric homopentameric protein, line shape analyses of CorA EPR spectra reveal the presence of strong spin–spin interaction at residues facing the five-fold symmetry axis along the pore [17] . Any movement that alters the intersubunit proximity would generate changes in the spin–spin coupling of spatially close residues (≤15 Å). Because of the complications owing to the distance relations in a pentameric geometry, we have estimated the intersubunit relative proximity from the ratio of the normalized amplitude of the spectra in the open and closed conformation (the Ω parameter adapted from Perozo et al. [27] , see Methods section). Negative Ω values indicate that the labelled positions are moving closer to the five-fold axis of symmetry, whereas positive Ω values reflect motion away from the symmetry axis. Plotting the Ω values versus the residue sequence revealed that residues at the tip of the C-terminal end of the stalk helix move closer to the symmetry axis as the channel opens ( Fig. 5a,b ). Beyond residue Asp270, the vast majority of the positions move further away from the centre, indicating an expansion of the cavity and permeation path ( Fig. 5b ). In the closed conformation structure, we and others have shown that permeation of a point charge through CorA is limited by several energy barriers along the permeation pathway [16] , [17] . Any conformational change triggering CorA opening must lower the amplitude of these barriers. Considering the presence of a kink in the stalk helix at position Gly273 and a pivot point, it is conceivable that a closure of the tip of the stalk helix would translate into an expansion of the funnel and the permeation pathway ( Supplementary Fig. 3 ). Dipolar coupling at positions flanking the constricted permeation pathway clearly indicate the dilation of the permeation pathway throughout its length, supporting the idea of an open channel ( Supplementary Fig. 4 ). 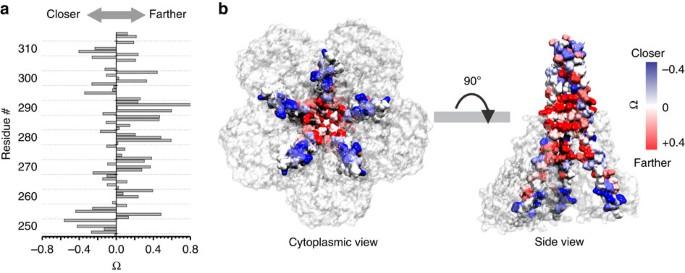Figure 5: Change in intersubunit proximities in the Stalk and in the pore-forming TM1 helices. (a) The bars represent the Ω parameter that reports on the relative intersubunit proximity change when the channel goes from the closed to the open state. Ω is defined by the ratio of the intensities of the central resonance line of the EPR spectra for the same sample in presence of 20 mM Mg2+and in absence of Mg2+(see Methods section). (b) Ω values are colour scaled and mapped on the CorA crystal structure (closed conformation). Two views are presented and for clarity purposes TM2 has been removed and on the side view one subunit has been removed so the pore-facing residues are visible. Figure 5: Change in intersubunit proximities in the Stalk and in the pore-forming TM1 helices. ( a ) The bars represent the Ω parameter that reports on the relative intersubunit proximity change when the channel goes from the closed to the open state. Ω is defined by the ratio of the intensities of the central resonance line of the EPR spectra for the same sample in presence of 20 mM Mg 2+ and in absence of Mg 2+ (see Methods section). ( b ) Ω values are colour scaled and mapped on the CorA crystal structure (closed conformation). Two views are presented and for clarity purposes TM2 has been removed and on the side view one subunit has been removed so the pore-facing residues are visible. Full size image This type of structural rearrangement is incompatible with a classical transporter-like mechanism where the protein alters its conformation from an inward facing to outward facing conformation by means of a rocking motion. This interpretation is also supported by the anomalous mole fraction effect observed in Ni 2+ / Mg 2+ mixtures, indicating that CorA pore is multi-occupied [13] . Our results are also consistent with MD simulations data suggesting an iris-like mechanism of opening [16] . To quantify the amplitude of the motion described above, we carried out double electron-electron resonance (DEER) spectroscopy experiments to calculate the average distances and distance distributions of interprobe distances [28] under different Mg 2+ concentrations. Recently, we have shown that using a symmetry-based constraints fit, we can accurately measure distance distributions on homomeric proteins [29] . Labelling positions at residues Thr247, Pro249, Tyr250 and Arg252 were selected to be within the working distance range of the DEER technique (20–70 Å). 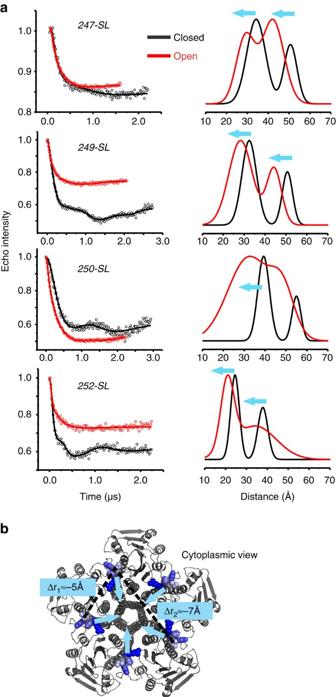Figure 6: Quantification of the stalk helix inward motion by DEER spectroscopy. (a) Background-corrected dipolar evolutions are shown as open circles for four different mutants. The fitted data are represented as solid lines and the corresponding distance distributions are illustrated using the same colour code. (b) The labelled positions are shown in blue on the cytoplasmic view of CorA crystal structures. Two dotted line represent the adjacent <r1> and the diagonal <r2> components of the distance distribution and the blue arrows schematize the inferred motion. Figure 6 shows that for the four positions at the end of the stalk helix, both the short adjacent and the long diagonal distance in the pentamer decrease ~5 Å when the open state is populated ( Supplementary Table 1 ). These measurements describe a relatively large closure movement of the stalk helix upon gating ( Fig. 6b ). The larger amplitude of the distance distribution in the open channel is compatible with an increase of protein dynamics that could interfere with the crystallization of this conductive conformation [14] . Such a movement is likely to dampen away from the hinge point and is expected to produce sufficient torque to propagate into the permeation pathway (TM1), generating the relatively large pore widening suggested above on the basis of the changes in environmental parameters ( Fig. 4 ). Figure 6: Quantification of the stalk helix inward motion by DEER spectroscopy. ( a ) Background-corrected dipolar evolutions are shown as open circles for four different mutants. The fitted data are represented as solid lines and the corresponding distance distributions are illustrated using the same colour code. ( b ) The labelled positions are shown in blue on the cytoplasmic view of CorA crystal structures. Two dotted line represent the adjacent <r 1 > and the diagonal <r 2 > components of the distance distribution and the blue arrows schematize the inferred motion. Full size image A model of CorA in its open conformation We have taken advantage of the present set of structural data as constraints to build 3D models of CorA in its open conformation. Accessibility data together with intersubunit distance changes were applied to the existing ‘closed’ conformation structure (Mg 2+ -bound) by means of restrained MD simulation using solvent accessibility as a soft constraint [30] ( Fig. 7 and Supplementary Figs 6 and 7 ). Model generation was limited to the regions of CorA from which experimental data is available, including the long stalk helix, the TM helices and the extracellular loop. The accessibility restraints were enforced through Lennard–Jones-like interactions between a pseudoatom representation of the SL and environmental probe-surrounding particles [30] ( Fig. 7a ). Intersubunit Cβ–Cβ distances estimated from DEER experiments, together with the accessibility data, were used to generate multiple models by varying the distance constraint boundary, increasing MD refining cycles and replicating the pentamer structure from individual subunits ( Supplementary Table 2 ). After validation, the top 25 models were subsequently refined using the accessibility restraints ( Fig. 7b and Supplementary Fig. 7 ). After a second round of refinement, the top 10 models show good structural convergence with a root mean square difference (RMSD) of 2.12±0.54 Å of each other ( Fig. 7c ). The stability of the top-ranked structure was evaluated by an all-atom MD simulation in a fully hydrated phospholipid bilayer. After 5 ns of simulation, the stalk and inner helices are stable ~3–5 Å RMSD from the starting structure for the whole-simulated time (25 ns) ( Supplementary Fig. 8 ). From the simulations, few transient changes in secondary structure of the open model are observed but the overall secondary pattern of the open model is similar to that of the closed structure ( Fig. 7d ). This suggests that the open model is a plausible structure for CorA in its open conformation. 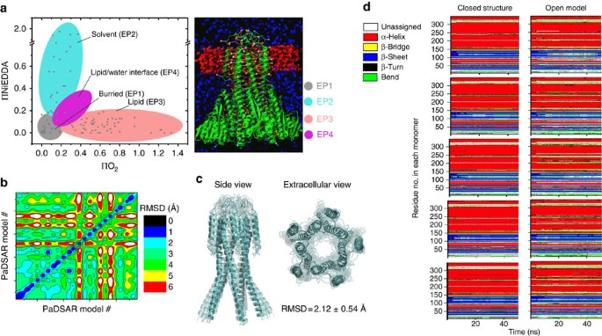Figure 7: Structural model building and validation for CorA in its open conformation. (a) PaDSAR translates solvent accessibility into structural restraints30(for details see Methods section andSupplementary Fig. 6). The pseudoatom probes are classified in four categories according to their EPR environmental parameters (left panel) and the starting structure (right panel) is equilibrated into a slab of O2molecules, representing the lipid bilayer (red spheres). NiEDDA relaxing agent is represented by blue spheres. (b) Hundreds of models were generated and evaluated according to their agreement with experimental data (Supplementary Fig. 7). The 25 best models candidates were selected for a second round of PaDSAR refinement and the pairwise Cα-RMSD matrix of the 25 PaDSAR models are colour scaled and coded on the contour plot. (c) An ensemble of 10 models show strong converging structures with backbone RMSD of 2.1 Å±0.5 for the regions where EPR data were obtained. (d) An all-atoms MD simulations of closed and open CorA embedded in a hydrated lipid bilayer was performed. Secondary structure elements were assigned according to DSSP algorithm52. Stability of the closed and open structures secondary structure elements was followed during the time course of the unrestrained MD simulation. The residue run from 6 to 349 are coloured coded depending on their secondary structure as followed: α-helix (red), stand in β-sheet (blue), β-bridge (yellow), β-turn (black), coil (green), unassigned (white). Figure 7: Structural model building and validation for CorA in its open conformation. ( a ) PaDSAR translates solvent accessibility into structural restraints [30] (for details see Methods section and Supplementary Fig. 6 ). The pseudoatom probes are classified in four categories according to their EPR environmental parameters (left panel) and the starting structure (right panel) is equilibrated into a slab of O 2 molecules, representing the lipid bilayer (red spheres). NiEDDA relaxing agent is represented by blue spheres. ( b ) Hundreds of models were generated and evaluated according to their agreement with experimental data ( Supplementary Fig. 7 ). The 25 best models candidates were selected for a second round of PaDSAR refinement and the pairwise Cα-RMSD matrix of the 25 PaDSAR models are colour scaled and coded on the contour plot. ( c ) An ensemble of 10 models show strong converging structures with backbone RMSD of 2.1 Å±0.5 for the regions where EPR data were obtained. ( d ) An all-atoms MD simulations of closed and open CorA embedded in a hydrated lipid bilayer was performed. Secondary structure elements were assigned according to DSSP algorithm [52] . Stability of the closed and open structures secondary structure elements was followed during the time course of the unrestrained MD simulation. The residue run from 6 to 349 are coloured coded depending on their secondary structure as followed: α-helix (red), stand in β-sheet (blue), β-bridge (yellow), β-turn (black), coil (green), unassigned (white). Full size image Superimposing the two CorA permeation pathway models offers a glimpse of the nature and extent of the conformational transition taking place during Mg 2+ -driven gating ( Fig. 8 ). The tips of the stalk helix come together towards the axis of symmetry like the nozzle of a jet-engine. After a kink, this motion translates into an expansion of the cavity and the mouth of the pore opens up with a motion reminiscent of an iris of a camera. These conformational transitions are best appreciated by observing the linear interpolation between the two states and illustrates the negative feedback mechanism first anticipated by Maguire and colleagues [5] , [6] , [7] ( Supplementary movie ). Given the low resolution of our spectroscopic approach, we choose to analyse the pore radius profile of our 10 best-ranked models ( Fig. 8b ). The comparison of the two conformational states clearly indicates a pore expansion throughout the length of the permeation pathway. Interestingly, the expansion is relatively modest on the upper part of the pathway around the signature sequence residues, consistent with their putative participation in Mg 2+ selectivity [14] , [18] . The pore dilation is larger (+5 Å) for the most constricted region of the pore, especially for the hydrophobic gates formed by Met292 and Leu294. These increases in the pore radius profile are consistent with expectations for an open channel, and suggest that our average model represents a plausible structure for the conductive state of CorA. Poisson–Boltzmann (PB) electrostatic calculation performed on our 10 best-ranked models shows that the large energy barriers impeding ion conduction in the closed state are largely alleviated ( Supplementary Fig. 9 ). Altogether, our results support an explicit molecular mechanism of magnesium regulation in prokaryotes where CorA acts as a Mg 2+ -deactivated Mg 2+ -selective channel as part of an homeostatic negative feedback loop ( Fig. 8c ). 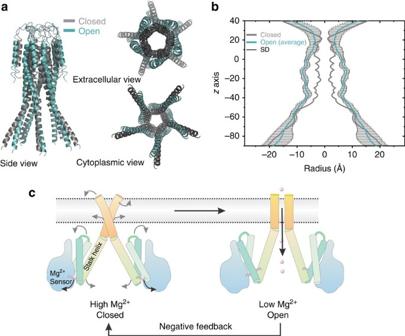Figure 8: Mg2+-dependent gating mechanism of CorA. (a) The open model generated by restrained MD simulation is shown in teal and the closed-state crystal structure is shown as grey cartoon. Only the positions measured by EPR are shown. (b) The pore radius profile was calculated for our 10 best-ranked open models using the program HOLE40. The average value is plotted in teal colour and the s.d. values are plotted in black. The profile for the closed structure is plotted in grey colour for comparison. (c) Cartoon summarizing the structural rearrangements is associated with the Mg2+-gating process regulating closing and opening of CorA. When the intracellular [Mg2+] drops below 2 mM, Mg2+leaves its regulatory-binding site, triggering a closing motion of the stalk helix. This motion propagates as a widening of the permeation pathway switching the conformation to a conductive state. Figure 8: Mg 2+ -dependent gating mechanism of CorA. ( a ) The open model generated by restrained MD simulation is shown in teal and the closed-state crystal structure is shown as grey cartoon. Only the positions measured by EPR are shown. ( b ) The pore radius profile was calculated for our 10 best-ranked open models using the program HOLE [40] . The average value is plotted in teal colour and the s.d. values are plotted in black. The profile for the closed structure is plotted in grey colour for comparison. ( c ) Cartoon summarizing the structural rearrangements is associated with the Mg 2+ -gating process regulating closing and opening of CorA. When the intracellular [Mg 2+ ] drops below 2 mM, Mg 2+ leaves its regulatory-binding site, triggering a closing motion of the stalk helix. This motion propagates as a widening of the permeation pathway switching the conformation to a conductive state. Full size image Molecular biology and Xenopus laevis oocyte overexpression CorA from T. maritima was sub-cloned in the pbstA vector optimized for oocyte expression [31] using the unique restriction sites NcoI and Xba1 and the PCR primers 5′-AAAAACCATGGAGGAAAAGAGGCTGTCTGCT-3′ and 5′-AAAAATCTAGATTAGAGCCACTTCTTTTTCTTGAA-3′. For expression assay only, the same gene was cloned in C-terminal fusion with Venus, a brighter version of the fluorescent protein YFP [32] using the primers 5′-AAAAAACTAGTATGGGCAGCAGCCATCATCATCAT-3′ and 5′-AAAAATCTAGATTAGAGCCACTTCTTTTTCTTGAA-3′ and unique restriction site SpeI and XbaI. Expression was monitored after 24 and 48 h of injection by confocal microscopy on an Olympus DSU Spinning Disk Confocal microscope on oocyte injected with constructs and with blank as control. Mutations were introduced by PCR using mismatch mutagenic primers as described by the Stratagene Quick Change kit. All mutant plasmid were amplified in Escherichia. coli XL-1 Blue Strain and purified by Mini or Midi Prep kit (Qiagen) and verified by whole-gene sequencing. Plasmid DNA (10 μg) were linearized by overnight Not1 digestion, verified by 1% agarose electrophoresis and purified by the QIAquick PCR purification (Qiagen) following the suppliers recommendation. Purified linear DNA (1 μg) was used as template for in vitro transcription (Ambion) and after purification the RNA were aliquoted and kept frozen at −80 °C. Oocyte were harvested from survival surgery on adult frog according to standard protocol and injected with 50 ng of mRNA. Electrophysiology Electrophysiology measurements were performed on custom-made two-electrode voltage clamp setups according to basic standards procedure [33] . The external solutions were isosmotic and typically composed by Hepes/ N -methyl-D-gluconamide (NMG) 10 mM, NMG-methanesulfonic acid, 30 mM NMG-Cl and 20 mM MgCl 2 . The cut-open oocyte preparation was used in experiments requiring control of intracellular [Mg 2+ ]. This consisted of a Vaseline-gap oocyte chamber following the original design of Perozo et al. [34] , where an internal perfusion cannula runs through the internal and guard compartments using a small stainless steel needle (33 gauge) connected to a syringe pump. After mounting the oocyte in the chamber, a micro needle was inserted midway through the bottom of the oocyte and perfusion was begun with internal solution buffered with a mixture of EDTA/EGTA. Internal Mg 2+ was successively increased from 0 to 2, 4, 40 and 60 mM by changing the internal perfusion solution. The internal perfusion rate was constant at 10 μl h −1 , and 10–15 min was required for equilibration at each new internal [Mg 2+ ]. Sample preparation and CW-EPR spectroscopy Cysteine mutants were expressed in E. coli BL21DE3-pLysS strain as previously described [17] . Immediately after elution from the Co 2+ column, the purified protein were reacted with a 10 molar excess of SL for 30 min on ice, followed by second addition of 10 molar probe excess and reacted for an additional 30 min. The reaction was stopped by addition of 1,000-fold excess of L-cysteine and the excess probe was removed by gel filtration chromatography. Reconstitution was carried out by destabilizing the pre-formed 1-palmitoyl-2-oleoyl-sn-glycerol-3-phosphatidylcholine (POPC)–POPG 3:1 liposomes with a saturating concentration of Triton X-100 (0.2 (w/w) ratio) before adding labelled protein to the liposome suspension in a 1/1500 protein/lipid molar ratio. Detergent was removed by successive addition of Bio-Beads SM-2 (Bio-Rad) and proteoliposomes were harvested by ultracentrifugation at 200,000 g and resuspended into 200 μl. Samples were split into two and were equilibrated with a buffer containing either 1 mM EDTA or 20 mM MgCl 2 . CW-EPR spectroscopic measurements were performed at room temperature on a Bruker EMX X-band spectrometer equipped with a dielectric resonator (ER 4123D). SL samples were loaded into a gas-permeable TPX plastic capillary and spectra were recorded at 2.0 mW incident power, 100 kHz modulation frequency with 1.0 G of modulation amplitude. The motional freedom of the SL was quantified as a peak-to-peak first-derivative width of the central resonance line ( ) [22] . Solvent exposure was measured form power-saturation experiments in which the vertical peak-to-peak amplitude of the central line of the EPR spectra is measured as a function of increasing incident microwave power [25] , [26] . Prior and during the recording of the spectra the sample are equilibrated with N 2 , air (20% O 2 ) or with 25 mM NiEDDA (Ni[II]ethylenediaminediacetic acid) in presence of N 2 . Accessibility parameters П were calculated as described in a previous report [17] . High accessibility of the spin probe to O 2 is witnessed by a high value of the ΠO 2 and is diagnostic of a membrane exposed residue, whereas high NiEDDA accessibility (ΠNiEDDA) is diagnostic of a water-exposed residue. The relative probe proximity change was determined by calculating the Ω parameter. The Ω parameter is defined by the ratio of the intensities of the central resonance line M =0 for the same sample exposed in two different experimental conditions as followed: where is the amplitude of M =0 measured in absence of Mg 2+ (open conformation) and is the amplitude of M =0 measured in presence of 20 mM Mg 2+ (closed conformation). We shifted the axis with the operator −1 to scale the values for negative/positive values instead of below/above 1. DEER experiments Samples concentration was empirically optimized to 75 μM of CorA pentamer and were loaded into a quartz capillary (Vitrocom) and equilibrated at 80 K under a flow of liquid N 2 using an Oxford cryostat. A standard four-pulse DEER sequence was conducted on a Bruker Elexsys 580 EPR spectrometer equipped with a 3-mm split-ring resonator. The four-pulse DEER sequence was set with pulses of 16 ns (90°) and 32 ns (180°), and evolution times were typically set to 1,800–2,500 ns depending on distance and signal quality. Refocused echo intensity evolutions were recorded, and these phase-corrected signals were background-corrected assuming a homogeneous 3D distribution ( Supplementary Fig. 5 ). The distance distribution P(r) was recovered from DEER measurements by a model fit of a two-component Rice 3D mixture with distance ratio constraint using 1.578< k <1.645 as determined from our previous study [29] . Analysis was performed on a modified version of DeerAnalysis 2011 programme [35] . Each time domain dipolar evolution data set was preprocessed using tools provided by DeerAnalysis to correct for experimental phase errors and to separate the intramolecular distances from the intermolecular background contribution. The background was assumed as a homogeneous distribution in three dimensions, appropriate for SL membrane proteins in detergent micelles. Molecular modelling The starting structure of CorA was taken from our previous work [17] . As mentioned previously, this model of the closed state of CorA was derived from the crystal structure (PDB 2UIB) with remodelling of the unresolved loop (residues 315–325). The structure of CorA is a homopentamer with 344 amino-acid residues per monomer starting from residues 6 to 349. For the calculation of the CorA open model, we used our previously developed method called PaDSAR (pseudoatom driven solvent accessibility refinement), restrained MDs using EPR accessibility restraints [30] . For the present work, the PaDSAR method has been incorporated in CHARMM c35b6 (ref. 36 ). Two sources of experimentally based restraints used in PaDSAR are the interprobe distances and solvent accessibility data. The detailed method is described below. Analyses of intersubunit DEER distances and the proximity profile of the open and closed states of CorA allow one to estimate a range of distance changes of the labelled positions at the backbone level. In the structure calculation, distance restraints ( ) were defined as a distance difference between intersubunit Cβ-positions of the labelled residues measured between the candidate open model and the closed-state X-ray structure as follow: where i is the residue number, of which the experimentally derived distance accounted for the following residue pairs: 247–247′, 249–249′, 250–250′ and 252–252′ (the prime is used to denote different subunits). As a pentameric protein, the ‘short’ and ‘long’ distance restraints were used to keep five subunits arranged about a five-fold symmetry axis. The short distance defined an intersubunit Cβ–Cβ separation of the residue between a subunit and its first adjacent subunit. whereas the long distance defined that of the residue between a subunit and its second adjacent subunit. From experimental data, the short and long distance restraints were set to −5± δ Å and −7± δ Å, respectively. The negative value of distance indicates that the residue pair of an expected open model is getting closer with respect to that of the closed-state structure. The δ values were used to define the upper and lower bound. A list of the intersubunit Cβ–Cβ distance restraints used in the calculations is given in Supplementary Table 2 . The accessibility restraints used in PaDSAR were derived from the experimental ПO 2 and ПNiEDDA accessibility data of more than 100 SL CorA mutants. The SL-positions covered a broad region of the protein domain including the long stalk helix (residues 246–293), the pore-forming TM1 helix (residues 294–314), the extracellular loop (residues 315–325) and the lipid-facing TM2 helix (residues 326–348). The restraints are described in terms of the Lennard–Jones-like interactions between various types of spin probe pseudoatoms attached to the Cα-atom of protein backbone and the surrounding environment pseudoatoms presented by OXY (O 2 ), NIC (NiEDDA) or PROT (amino-acid residue). In the calculation, four types of the spin pseudoatoms ( Fig. 7 and Supplementary Fig. 6 ) have first been assigned to individual SL-residue of CorA before the PaDSAR calculation. The assignment was on the basis of residue-based surface exposure from an analysis of ΠO 2 , ΠNiEDDA and ΔH o -1 profiles. An initial configuration of modelling system comprising the starting structure of the CorA pentamer attached with the 83 assigned spin pseudoatoms and several hundreds of OXY and NIC pseudoatoms is illustrated in Fig. 7a . The modelling of the CorA open structure may be divided into two main PaDSAR runs. The first run was carried out using the delta distance (Δ r CB ) and accessibility restraints imposed on the starting structure as described in previous section. The protein was modelled with the united-atom CHARMM PARAM19 force field [37] . During the calculation, we restrained the N-terminal domain (residues 6–156) and secondary structures including residues 165–199, 204–237, 243–310 (stalk and TM1 helices) and 327–347 (TM2 helix). OXY and NIC pseudoatoms move within a defined boundary using the miscellaneous mean field potential in CHARMM [38] . OXY pseudoatoms were allowed to move in the membrane region, whereas NIC pseudoatoms were distributed outside the membrane but within the defined boundary ( Supplementary Fig. 6 ). We varied the upper and lower bound of distance restraints ( δ =1 and 2) and increased MD refining cycles to generate a set of model candidates. However, it appears that these model candidates tend to lose their five-fold symmetry. Therefore, we took an individual subunit of all the resulting models and replicated their own pentamer structure. As a result, hundreds of model candidates were generated, and subsequently evaluated by considering with the following experimental-based validation: (1) the restraint penalty ( P rstrnt ) and distance restraint violation ( viol ) [39] , and (2) a consensus change between the evaluated model and the intersubunit proximity (Ω). For the former validation, P rstrnt is given as where and are the upper and lower distance restraints, and k rstrnt is an arbitrary constant value. The latter validation was made by identifying the closer or further Cβ–Cβ distance of individual SL residues (the short distance or first adjacent subunit) with respect to the closed-state conformation and comparing with the positive or negative signs of Ω parameters ( Fig. 5 ). The best-fit 25 models selected based on an averaged fit criterion were subjected to structure refinement of the PaDSAR run. In the second run, the top 25 models were refined using the accessibility restraint only. Similar protocol of PaDSAR refinement described above, except no distance restraint was imposed at this step. In addition, PaDSAR treated each model as a single subunit, and refined it using the image facility within the CHARMM programme to maintain the five-fold symmetry of the CorA pentamer. In addition to the model validation described previously, inspections of the resulting structures obtained in the second run include structure convergence (RMSD), the HOLE plot [40] , the accessibility mapped molecular surface and all-atom MD simulations. Model validation by PB energy calculation of ion translocation Model quality was assessed by calculating the solvation-free energy profile of ion translocation along the permeation pathway. We used PB continuum method to compute free-energy barrier for Mg 2+ translocation through the CorA tranmembrane pore of the closed and open conformations. The PB calculation was performed using Adaptive PB Solver (APBS) [41] . The programme PDB2PQR was used to add hydrogen atoms and assign atomic charges and radii to each generated configuration [42] , [43] . Partial atomic charges and radii of the protein were taken from the CHARMM parameter sets [44] . The CorA protein was oriented with its symmetry axis coinciding with the z axis. The sequential focusing multigrid algorithm in solving PB equation consists of the following three resolution maps: 300 × 300 × 300 Å 3 for coarse, 200 × 200 × 200 Å 3 for medium and 100 × 100 × 100 Å 3 for fine resolutions. Grid points of 161 × 161 × 161 were used to all maps. The implicit membrane hydrophobic slab was defined between z =±12 Å. This corresponds to the thickness of hydrophobic slab of 24 Å. The dielectric constants for protein, membrane and water were 2, 2 and 80, respectively [45] . Ionic strength was 0.15 M with coulomb charge +1 and −1, and radius 2.0 Å. Water probe radius was 1.4 Å. The solvation-free energy profile of Mg 2+ translocation through the TmCorA pore was computed by systematically varying Mg 2+ positions from z =+20 Å (periplasmic region) to z =−40 Å (cytoplasmic region) with 1 Å steps along the z axis. The program APBSmem was used to set up and to monitor the membrane region [46] . For each configuration, electrostatic contribution to the solvation-free energy was computed twice, one for implicit aqueous model and one for water-membrane model, giving rise to Δ G elec,water and Δ G elec,membrane , respectively. The solvation-free energy (ΔΔ G elec ) that is the electrostatic free-energy difference of the proteins embedded in the two solvent environments was obtained according to Equation (4) Model validation by explicit solvent MDs simulation An obtained model was subsequently inserted into a pre-equilibrated lipid bilayer, made up of ~480 molecules of POPC embedded in ~64,000 TIP3P waters. Side-chain ionization states that were expected at pH=7 were assigned based on pK a calculations using PROPKA [47] . Sodium and chloride counter ions were added to neutralize charges on the system using VMD’s Autoionize plugin [48] . Total number of atoms in the simulation is ~300,000 atoms. The MD simulations were carried out using NAMD 2.8b2 with the all-atoms CHARMM22 and CHARMM27 force fields for protein, lipid and ion [49] . The TIP3P models were used for waters. At this stage, the pseudoatoms present in the model were removed; no pseudoatom restraints were included during the simulation with explicit solvent models. To reduce finite-size effects, periodic boundary conditions were used in MDs simulations with a periodic dimension of 144x144 × 155 Å 3 . The calculation of long-rang electrostatic interactions in periodic membrane-protein system used the particle mesh Ewald summation via fast Fourier transform (FFT). The particle mesh Ewald grid size was set to at least one cell per Angstrom in each dimension. A distance cutoff of 12 Å was used with a switching distance set at 10 Å. The non-iterative SETTLE algorithm was used to keep waters rigid. Rigid bonds between the hydrogen and the heavy atom to which it is attached were enabled. The simulations were performed at constant pressure of 1 atm and constant temperature of 300 K. Langevin dynamics was used to keep a constant temperature of the system with Langevin damping coefficient of 1 ps −1 . The pressure of the system was controlled using a Nośe–Hoove Langevin Piston. Energy minimizations and restrained MD simulations were used to relax geometric, angle, torsional and other structural distortions restrains of the model systems. During the first restrained MD run, atoms for protein and lipid head groups were restrained to their initial positions using harmonic constraints with a force constant of 1 kcal mol −1 Å −2 . In the subsequent run, protein atoms were restrained, leaving the rest of the system to be relaxed. Finally, all positional restraints were removed and an equilibration run was performed. MD simulations were performed for 25 ns with the time step of 2 fs. The configurations and velocities were stored every 2 ps. The programs VMD, WORDOM [50] , DSSP [51] and APBS [41] , [46] were used for assessment of protein structure stability, RMSD and visualization. How to cite this article: Dalmas, O. et al. Molecular Mechanism of Mg 2+ -dependent gating in CorA. Nat. Commun. 5:3590 doi: 10.1038/ncomms4590 (2014).